Endopolyploidization and flowering time are antagonistically regulated by checkpoint component MAD1 and immunity modulator MOS1 The spindle assembly checkpoint complex (SAC) is essential for quality control during mitosis in yeast and animals. However, its function in plants is not well understood. Here we show that MAD1, an Arabidopsis SAC component, is involved in endopolyploidization and flowering time via genetic interaction with MOS1, a negative regulator of plant immunity. MOS1 is found to interact with MAD2, another SAC component, and promote flowering and inhibit endopolyploidization, but this function is antagonized by MAD1. Furthermore, MAD1 and MOS1 both interact with SUF4, a transcription factor regulating the expression of the flowering time gene FLC . These findings reveal MOS1, MAD1 and SUF4 as regulators of endopolyploidization and flowering time and suggest an involvement of cell cycle control in the timing of reproductive transition. In yeast and animal cells, spindle assembly checkpoint (SAC) acts as a safeguard to ensure the accurate cell cycle progression. SAC proteins include Mitotic Arrest Deficient (MAD) 1, 2 and 3 and Budding Unperturbed by Benzimidazole (Bub) 1, 2 and 3 (ref. 1 ). MAD1 is localized predominantly at unattached kinetochore and recruits MAD2 to form a MAD1–MAD2 complex. The closed form of MAD2 is bound to MAD1 and serves as a template for the conversion of the open form MAD2 into the closed form [2] . Closed MAD2 binds to CDC20 and the formation of MAD2–CDC20 complex promotes the binding of BUB3 and MAD3/BUB1-related 1 (BUBR1) to form mitotic checkpoint complex [3] , [4] . Functional mitotic checkpoint complex prevents aberrant chromosome segregation at mitosis until all chromosomes are properly attached to spindles. In maize, the MAD2 homologue was found to localize at the kinetochore and this localization was postulated to be sensitive to microtubule attachment and tension, respectively, during mitosis and meiosis [5] . In Arabidopsis , the homologues of SAC components including MAD1, MAD2, BUB3.1 and BUBR1 have been identified. Physical interactions among Arabidopsis MAD1, MAD2, BUB3.1 and BUBR1 were revealed by yeast two-hybrid (Y2H) and/or bimolecular fluorescence complementation (BiFC) assays, and the dynamics of their localization at kinetochore during the cell division suggest that they may have a SAC function [6] , [7] , [8] . However, the petal-specific knockdown of MAD2 and BUBR1 in Arabidopsi s did not cause any defects in mitosis, although they resulted in reduced petal growth [9] . The loss–of-function (l-o-f) mutant mad2–2 did not exhibit any defects except for an arrested root growth [7] . Therefore, the biological function of plant SAC homologues is still unclear. Here we identified a role of Arabidopsis MAD1 in flowering time and endopolyploidization control. Plants have a complex network to sense endogenous signals and environmental cues to ensure proper flowering time for reproductive success. At least four major pathways have been identified in floral transition control: photoperiod, autonomous, vernalization and gibberellin pathways [10] . Both the autonomous and vernalization pathways target the expression of the central flowering time gene FLC through chromatin remodelling [10] , [11] , [12] . SUF4 (Suppressor of FRIGIDA 4), a C2H2-type zinc-finger protein, is a transcriptional activator that binds to a cis-element of the FLC promoter [13] , [14] . It recruits EFS (EARLY FLOWERING IN SHORT DAYS) and PAF1 (RNA polymerase II-associated factor 1)-like complex to the FLC locus and induces histone H3 lysine 4 (H3K4) trimethylation to activate FLC expression [15] . In this study, we found that the Arabidopsis MAD1 interacts with MOS1 (MODIFIER OF snc1, 1), a regulator of plant immunity and flowering time [16] , [17] . We present evidence that MOS1 and MAD1 antagonistically regulate endopolyploidization and floral transition and these regulations are likely mediated by SUF4. These findings reveal a function of SAC in the control of endopolyploidization and flowering time and suggest an involvement of cell cycle control in reproductive transition. Loss of MOS1 function suppresses an autoimmune phenotype We isolated sbo3 ( suppressor of bon1-1 3) as a suppressor of the autoimmune mutant bon1-1 from a genetic screen. The bon1-1 (referred as bon1 ) plants were dwarf and had curly leaves due to the constitutive defense response induced by upregulation of an immune receptor gene SNC1 (refs 18 , 19 , 20 ). The sbo3 mutation suppressed the defects of both plant growth and disease resistance in bon1 ( Fig. 1a ). The virulent bacterial pathogen Pseudomonas syringae pv. tomato ( Pst ) DC3000 grew 10-fold more in sbo3 bon1 than in bon1 ( Fig. 1b ), and the expression of PR1 was dramatically reduced in sbo3 bon1 compared with bon1 as analysed by RNA blotting ( Fig. 1c ). Furthermore, an increase of SNC1 expression in bon1 was suppressed by the sbo3 mutation, indicating that SBO3 is required for SNC1 upregulation and its induced autoimmune response ( Fig. 1c ). 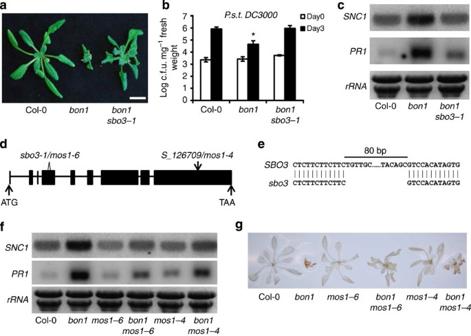Figure 1: Characterization of thesbo3mutation. (a) Morphology of Col-0,bon1andbon1 sbo3plants grown at 22 °C for 3 weeks. Scale bar, 1 cm. (b) Growth of virulent bacterial pathogenPseudomonas syringaepv.tomato(Pst) DC3000 in Col-0,bon1andbon1 sbo3at days 0 3 after inoculation. The error bars indicate s.d. determined from three replicates. The asterisk indicates a statistically significant difference from Col-0 determined by Student’st-test (P<0.05). (c) Expression ofSNC1andPR1genes in Col-0,bon1andbon1 sbo3as analysed by RNA blotting.rRNAs were used as loading controls. (d) Gene structure and mutations ofMOS1. A deletion mutation inmos1–6and a T-DNA insertion inmos1–4are indicated. (e) The DNA sequence flanking the 80-bp deletion inmos1–6. (f) Expression ofSNC1andPR1genes in indicated genotypes were analysed by RNA blotting.rRNAs were used as loading controls. (g) H2O2accumulation in the above genotypes analysed by DAB staining. Figure 1: Characterization of the sbo3 mutation. ( a ) Morphology of Col-0, bon1 and bon1 sbo3 plants grown at 22 °C for 3 weeks. Scale bar, 1 cm. ( b ) Growth of virulent bacterial pathogen Pseudomonas syringae pv. tomato ( Pst ) DC3000 in Col-0, bon1 and bon1 sbo3 at days 0 3 after inoculation. The error bars indicate s.d. determined from three replicates. The asterisk indicates a statistically significant difference from Col-0 determined by Student’s t -test ( P <0.05). ( c ) Expression of SNC1 and PR1 genes in Col-0, bon1 and bon1 sbo3 as analysed by RNA blotting. rRNA s were used as loading controls. ( d ) Gene structure and mutations of MOS1 . A deletion mutation in mos1–6 and a T-DNA insertion in mos1–4 are indicated. ( e ) The DNA sequence flanking the 80-bp deletion in mos1–6 . ( f ) Expression of SNC1 and PR1 genes in indicated genotypes were analysed by RNA blotting. rRNA s were used as loading controls. ( g ) H 2 O 2 accumulation in the above genotypes analysed by DAB staining. Full size image We identified the SBO3 gene as MOS1 through map-based cloning ( Supplementary Fig. 1a ) and sbo3 has an 80-bp deletion in the fourth exon of MOS1 ( Fig. 1d,e ). The identity of SBO3 was confirmed by complementing sbo3 with the wild-type MOS1 gene and the suppression of the bon1 phenotypes by a second allele of MOS1 , mos1–4 (Salk_126709) ( Supplementary Fig. 1b,c ). We thus named sbo3 as mos1–6 . The mos1–6 mutation has a stronger bon1 suppression effect than the mos1–4 mutation from a T-DNA insertion in the last exon of MOS1 . RNA blot analysis indicated that expression of both SNC1 and PR1 were more reduced in bon1 mos1–6 than in bon1 mos1–4 compared with bon1 ( Fig. 1f ). In addition, DAB (3,3′-Diaminobenzidine) staining was more pronouncedly reduced in the bon1 mos1–6 mutant ( Fig. 1g ), indicating that elevation of H 2 O 2 production in bon1 was more suppressed by the mos1–6 mutation than the mos1–4 mutation. Expression of the MOS1 gene and the MOS1 protein We determined MOS1 RNA expression pattern using its promoter and its first exon to control the expression of a reporter gene encoding GUS (β-glucuronidase). Consistent with microarray data ( www.genevestigator.com/gv/ ), this GUS reporter was expressed ubiquitously, including shoot apical meristem, root, hypocotyl, cotyledons and leaves ( Supplementary Fig. 2a ). MOS1 was previously reported to be expressed only in shoot meristems [16] , [17] , which might have resulted from a shorter regulatory sequence used in the reporter construct than in this study. We determined the subcellular localization of full-length MOS1 by expressing a green fluorescent protein (GFP) and MOS1 fusion under the control of the 35S promoter of cauliflower mosaic virus. This GFP:MOS1 fusion is functional as it complemented the mos1–6 mutation in bon1 ( Supplementary Fig. 2b ). In bon1 mos1–6 transgenic plants with the GFP:MOS1 fusion, weak GFP signals could be detected in young roots where autofluorescence is relatively low, and these signals appeared to be nuclear. The GFP:MOS1 signals were observed in the differentiation zone but not in the root tip or the elongation zone ( Supplementary Fig. 2c,d ). Treatment of roots with the proteasome inhibitor MG132 significantly increased MOS1 signals in the root tip and elongation zone ( Supplementary Fig. 2e,f ), indicating that the MOS1 protein could be degraded by the 26S proteasome in some tissues. When the MOS1 protein was transiently expressed in Nicotiana benthamiana , it was also found to be unstable. Western blot revealed multiple bands of MOS1 at sizes smaller than the expected full-length size, suggesting a protein degradation of MOS1 ( Supplementary Fig. 2g ). Therefore, the MOS1 protein is subject to degradation both in the transient expression system and transgenic plants. Taken together, MOS1 is transcribed ubiquitously but its protein is quickly turned over in a tissue- and development-dependent manner. MOS1 and MAD1 both interact with SUF4 A co-immunoprecipitation study identified MOS1 as an interactor of the Arabidopsis SAC component MAD2 in a large-scale co-IP screen on cell cycle regulators [8] . MAD2 could interact with other SAC components including MAD1 and BUB3.1 (refs 6 , 7 , 8 ). Intriguingly, SUF4, a flowering time regulator, was found to interact with BUB3.1 interacting protein in this screen [8] . Because the mos1 mutant was reported to have a late flowering time phenotype, we tested the interaction among MOS1, MAD2, MAD1, BUB3.1 and SUF4 using the GAL4-based Y2H systems. Positive interactions were found between MOS1 and MAD2 as well as between BUB3.1 and SUF4, while no interaction was observed between MOS1 and MAD1 or MOS1 and BUB3.1 ( Supplementary Fig. 3a,b ). The interaction between MOS1 and SUF4 is weaker than that between MAD1 and SUF4 judged by the extent of yeast growth on selection plates ( Fig. 2a ). 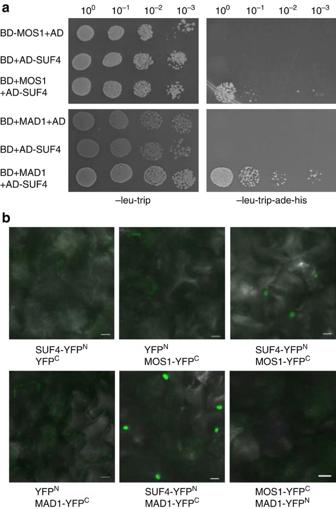Figure 2: Both MOS1 and MAD1 interact with SUF4. (a) Interactions between SUF4 and MOS1 and MAD1 analysed by Y2H. Shown are serial dilutions of yeast strains containing different combinations of constructs on the selection plate SC-Ade-His-Leu-Trp. AD: activation domain of GAL4. BD: DNA-binding domain of GAL4. (b) Confocal microscopy images from BiFC assay inN. benthamina. SUF4:YFPNtogether with MOS1:YFPCor MAD1:YFPCwere transiently expressed inN. benthamiana. Images were taken at 48 h after infiltration. Green signals are from YFP. Scale bar, 10 μm. Figure 2: Both MOS1 and MAD1 interact with SUF4. ( a ) Interactions between SUF4 and MOS1 and MAD1 analysed by Y2H. Shown are serial dilutions of yeast strains containing different combinations of constructs on the selection plate SC-Ade-His-Leu-Trp. AD: activation domain of GAL4. BD: DNA-binding domain of GAL4. ( b ) Confocal microscopy images from BiFC assay in N. benthamina . SUF4:YFP N together with MOS1:YFP C or MAD1:YFP C were transiently expressed in N. benthamiana . Images were taken at 48 h after infiltration. Green signals are from YFP. Scale bar, 10 μm. Full size image The interactions of MAD2 with MOS1, SUF4 with MOS1 and SUF4 with MAD1 were confirmed in planta by BiFC analysis [21] in Nicotiana benthamiana ( N. benthamiana ). The MAD2 and SUF4 protein was fused with the amino-terminal part of yellow fluorescent protein (YFP, MAD2-YFP N and SUF4-YFP N ), and MOS1 and MAD1 were, respectively, fused with the carboxyl-terminal part of YFP (MOS1-YFP C and MAD1-YFP C ). Co-expression of MAD2-YFP N and MOS1-YFP C generated fluorescence signals in the nucleus, and no signals were detected in controls with MOS1 or MAD2 co-expressing with a nuclear protein, OSD1 (Omission of Second Division 1; Supplementary Fig. 3c ). Co-expression of SUF4-YFP N with MOS1-YFP C or with MAD1-YFP C generated fluorescence signals in the nucleus, with MAD1-YFP C co-expression having a stronger signal than MOS1-YFP C co-expression ( Fig. 2b ). No signals were detected with co-expression of MOS1-YFP C with MAD1-YFP N ( Fig. 2b ), consistent with the observation from the Y2H assays. No signals were detected in the following co-expression controls: SUF4-YFP N with YFP C , YFP N with MOS1-YFP C , YFP N with MAD1-YFP C ( Fig. 2b ). These data indicate that MOS1 could physically interact with MAD2 and both MOS1 and MAD1 could interact with SUF4 in plants. MOS1 regulates floral transition through FLC The mos1–6 had a late flowering time phenotype, similar to what was reported for the mos1–4 mutant [17] ( Fig. 3a ). We found that the late flowering defect is due to an upregulation of FLC in the mos1 mutants. Vernalization, which reduces the FLC expression, suppressed the flowering defect in mos1 ( Fig. 3b ). Under a long-day growth condition (16 h light per day), mos1–6 had eight rosette leaves at bolting with vernalization (a 6-week 4 °C treatment) versus 14 rosette leaves without vernalization ( Fig. 3b ). FLC expression was elevated in both mos1–6 and mos1–4 mutants compared with the wild type as analysed by RT (reverse transcription)-PCR ( Fig. 3c ). Furthermore, the late flowering defect in mos1–6 is dependent on FLC ( Fig. 3d ). A l-o-f mutation flc-3 (ref. 22 ) was introduced into mos1–6 to generate the double mutant mos1–6 flc-3 . At bolting, the flc-3 mutant had 11 rosette leaves and mos1–6 had 17 leaves, both deviating from the 13 rosette leaves in Col-0. The mos1–6 flc-3 had 10 rosette leaves, similar to the flc-3 single mutant. Therefore, MOS1 promotes flowering through negatively regulating FLC . 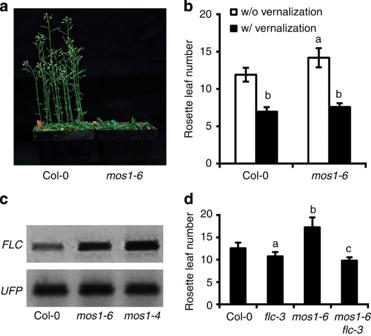Figure 3: Themos1mutations result in a late flowering phenotype. (a) Morphology of Col-0 andmos1–6plants grown for 4 weeks under constant light. (b) Comparison of flowering time in Col-0 andmos1–6grown under long-day growth condition (16 h light per day) with or without vernalization (6-week 4 °C treatment) (number of plants (n)>20). The letters a and b indicate statistically significant differences to various extents from Col-0 grown without vernalization determined by Student’st-test (P<0.05). (c) RT-PCR analysis ofFLCexpression in Col-0,mos1–6andmos1–4. (d) Comparison of flowering time in Col-0 (n=23),flc-3(n=25),mos1–6(n=25) andmos1–6 flc-3(n=25) grown under constant light. The letters a, b and c indicate statistically significant differences to various extents from Col-0 determined by Student’st-test (P<0.05). The error bars indicate s.d. Figure 3: The mos1 mutations result in a late flowering phenotype. ( a ) Morphology of Col-0 and mos1–6 plants grown for 4 weeks under constant light. ( b ) Comparison of flowering time in Col-0 and mos1–6 grown under long-day growth condition (16 h light per day) with or without vernalization (6-week 4 °C treatment) (number of plants ( n )>20). The letters a and b indicate statistically significant differences to various extents from Col-0 grown without vernalization determined by Student’s t -test ( P <0.05). ( c ) RT-PCR analysis of FLC expression in Col-0, mos1–6 and mos1–4 . ( d ) Comparison of flowering time in Col-0 ( n =23), flc-3 ( n =25), mos1–6 ( n =25) and mos1–6 flc-3 ( n =25) grown under constant light. The letters a, b and c indicate statistically significant differences to various extents from Col-0 determined by Student’s t -test ( P <0.05). The error bars indicate s.d. Full size image SUF4 mediates the flowering phenotype of mos1–6 To test the role of SUF4 in MOS1 -regulated flowering time, we introduced a SUF4 l-o-f mutation suf4–2 (ref. 15 ) into mos1–6 . While the suf4–2 mutation itself did not affect the flowering time, it abolished the late flowering phenotype of mos1–6 ( Fig. 4a ). At bolting, mos1–6 had 17 leaves, while mos1–6 suf4–2 had 13 rosette leaves similarly to suf4–2 and Col-0 ( Fig. 4b ). The suppression of late flowering is correlated with a reduction of FLC expression in mos1–6 suf4–2 . FLC had a decreased expression in suf4–2 than in Col-0 as analysed by RT-PCR ( Fig. 4c ), consistent with an earlier report [13] . Its expression was elevated in mos1–6 compared with Col-0, and this elevation was reduced in mos1–6 suf4–2 ( Fig. 4c ). Therefore, SUF4 is required for the FLC upregulation and late flowering defect in the mos1 mutant. 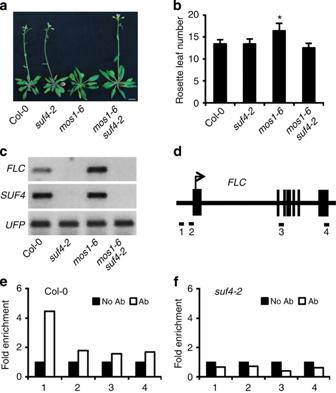Figure 4:MOS1-regulation of flowering time is dependent onSUF4. (a) Thesuf4–2mutation suppresses the late flowering phenotype ofmos1–6. Scale bar, 1 cm. (b) Comparison of flowering time in Col-0,suf4–2,mos1–6andmos1 suf4grown under constant light (n=15). The error bars indicate s.d. The asterisk indicates a statistically significant difference from Col-0 as determined by a Student’st-test (P<0.05). (c) RT-PCR analysis ofFLCexpression in Col-0,suf4–2, mos1–6andmos1–6 suf4–2. (d) Diagram of theFLCgene with four regions used for ChIP indicated (1, SUF4-binding site; 2,FLCTATA box; 3,FLCcoding; 4,FLCterminator)23. Black box indicates exons. (e,f) ChIP analysis of MOS1 association with different regions of theFLCgene in Col-0 (e) andsuf4–2(f). Shown is the enrichment of four regions of theFLCgene in samples precipitated with antibody (Ab) versus that without Ab analyzed by qPCR. The fold enrichment value is the average of two independent experiments. Figure 4: MOS1 -regulation of flowering time is dependent on SUF4 . ( a ) The suf4–2 mutation suppresses the late flowering phenotype of mos1–6 . Scale bar, 1 cm. ( b ) Comparison of flowering time in Col-0, suf4–2 , mos1–6 and mos1 suf4 grown under constant light ( n =15). The error bars indicate s.d. The asterisk indicates a statistically significant difference from Col-0 as determined by a Student’s t -test ( P <0.05). ( c ) RT-PCR analysis of FLC expression in Col-0, suf4–2, mos1–6 and mos1–6 suf4–2 . ( d ) Diagram of the FLC gene with four regions used for ChIP indicated (1, SUF4-binding site; 2, FLC TATA box; 3, FLC coding; 4, FLC terminator) [23] . Black box indicates exons. ( e , f ) ChIP analysis of MOS1 association with different regions of the FLC gene in Col-0 ( e ) and suf4–2 ( f ). Shown is the enrichment of four regions of the FLC gene in samples precipitated with antibody (Ab) versus that without Ab analyzed by qPCR. The fold enrichment value is the average of two independent experiments. Full size image We further tested the binding of the MOS1 protein to the FLC promoter and its dependence on SUF4 by chromatin immunoprecipitation (ChIP) in a protoplast expression system. The GFP–MOS1 fusion was transiently expressed under the strong 35S promoter in protoplasts isolated from the wild-type Col-0 and the suf4 mutant, respectively. Chromatin associated with GFP–MOS1 was precipitated with anti-GFP antibodies and four FLC genomic sites ( Fig. 4d ), including the SUF4-binding site [23] of the FLC promoter, were analysed for their abundance in the precipitated chromatins by quantitative (q)-PCR. Compared with the no antibody (Ab) IP sample, the Ab IP sample had a five-fold enrichment at the SUF4-binding site, while no significant enrichment was found at three other sites: TATA box, a coding fragment and the terminator ( Fig. 4e ). In addition, no enrichment of the Ab IP sample over the no Ab IP sample was observed in the suf4–2 mutant for any of the four sites including the SUF4 site ( Fig. 4f ). These data indicate that MOS1 is physically associated with the FLC promoter at or close to the SUF4-binding site, and this association is dependent on SUF4. MOS1 and MAD1 antagonistically regulate flowering time The association of SAC with MOS1 prompted us to analyse the role of SAC components in flowering time control. A mad2–2 mutant (SAIL_191_G06) [7] , and two mad1 mutants, mad1–1 (Salk_039008) and mad1–2 (Salk_073889), were isolated from the T-DNA insertion collection [24] , [25] ( Supplementary Fig. 4a,b ). Interestingly, both mad1–1 and mad1–2 mutants were slightly early in flowering than Col-0, with three fewer rosette leaves than Col-0 at bolting ( Fig. 5a,c ; Supplementary Fig. 4c ). Quantitative real-time RT-PCR (qRT-PCR) analysis revealed a 50% reduction of the FLC transcript in both mad1–1 and mad1–2 compared to the wild type, which is likely responsible for their early flowering phenotypes ( Fig. 5b ). The mos1–6 and mad1–1 single mutants bolted with 19 and 12 leaves, respectively, and the double mutant mos1–1 mad1–6 bolted with 16 leaves, approximately in between the single mutants ( Fig. 5c ). A slight but significant reduction of FLC transcript was detected in the mos1–6 mad1–1 double mutant compared with mos1–6 by qRT-PCR analysis ( Fig. 5d ). To further test the role of MAD1 in flowering time control through FLC , we introduced into the mad1–2 mutant a functional FRIGIDA ( FRI ) that induces a higher expression of FLC and consequently a late flowering phenotype in Col-0. Both the FRI and FRI mad1–2 plants were then grown at 22 °C for three weeks followed by 28 °C to accelerate flowering. The FRI plants bolted at 64 days under this condition, while FRI mad1–2 bolted earlier at 49 days ( Fig. 5e,f ). When grown constantly at 22 °C, the FRI mad1–2 plants bolted at 80 days, 20 days earlier than the FRI plants ( Fig. 5f ). Thus, MAD1 is a positive regulator of FLC in floral transition and this function is antagonistic to MOS1 . 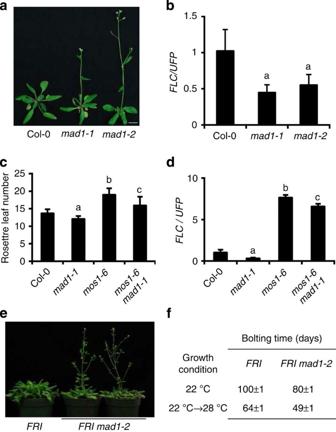Figure 5: MAD1 antagonizes MOS1 function on the flowering time regulation. (a) Morphology of Col-0,mad1–1andmad1–2plants grown for 4 weeks under constant light. Scale bar, 1 cm. (b) qRT-PCR analysis ofFLCexpression in Col-0,mad1–1andmad1–2. (c) Comparison of flowering time in Col-0 (n=23),mad1–1(n=18),mos1–6(13) andmos1 mad1(n=18) grown under constant light. The error bars indicate s.d. (d) qRT-PCR analysis ofFLCexpression in Col-0,mad1–1,mos1–6andmos1–6 mad1–1. (e) Morphology ofFRI(Col-0) andFRI mad1–2plants grown at 22 °C for the first 3 weeks and 5 weeks at 28 °C. (f) Bolting time ofFRI(Col-0) andFRI mad1–2plants grown at 22 °C only or 22 °C for 3 weeks followed by 28 °C. The error bars indicate s.d. determined from three measurements. The letters a, b and c indicate statistically significant differences from Col-0 determined by Student’st-test (P<0.05). Figure 5: MAD1 antagonizes MOS1 function on the flowering time regulation. ( a ) Morphology of Col-0, mad1–1 and mad1–2 plants grown for 4 weeks under constant light. Scale bar, 1 cm. ( b ) qRT-PCR analysis of FLC expression in Col-0, mad1–1 and mad1–2 . ( c ) Comparison of flowering time in Col-0 ( n =23), mad1–1 ( n =18), mos1–6 (13) and mos1 mad1 ( n =18) grown under constant light. The error bars indicate s.d. ( d ) qRT-PCR analysis of FLC expression in Col-0, mad1–1 , mos1–6 and mos1–6 mad1–1 . ( e ) Morphology of FRI (Col-0) and FRI mad1–2 plants grown at 22 °C for the first 3 weeks and 5 weeks at 28 °C. ( f ) Bolting time of FRI (Col-0) and FRI mad1–2 plants grown at 22 °C only or 22 °C for 3 weeks followed by 28 °C. The error bars indicate s.d. determined from three measurements. The letters a, b and c indicate statistically significant differences from Col-0 determined by Student’s t -test ( P <0.05). Full size image MOS1 and MAD1 affect endopolyploidization and cell size The interaction between MOS1 and a SAC component prompted us to investigate the potential effects of mos1 mutations on cell cycle progression. Ploidy distribution among cells was measured in the first pair of leaves from 3-week-old plants using a flow cytometer ( Fig. 6a ). In mos1–6 and mos1–4 , the portion of 16C cells increased to 30 and 28%, respectively, from 22% in Col-0. The portion of 8C cells decreased from 48% in Col-0 to 38% in mos1–6 and 40% in mos1–4 . Correspondingly, the mos1 mutants had significantly higher ploidy indices, at 2.99 for mos1–6 and 2.94 for mos1–4 compared with 2.80 in Col-0 ( Fig. 6a ). Thus, both mos1 mutations result in an enhanced endopolyploidization with mos1–6 having a stronger effect than mos1–4 . 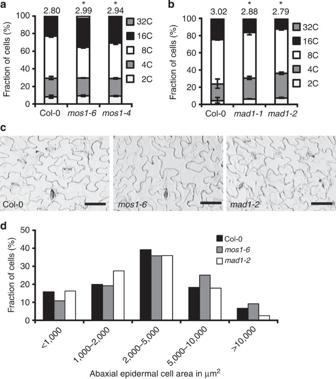Figure 6: MOS1 and MAD1 affect endopolyploidization in an opposite manner. (a,b) Ploidy levels in the first pair of leaves from (a) the wild-type Col-0,mos1–6andmos1–4and (b) Col-0,mad1–1andmad1–2. The error bars indicate s.d. determined from three replicates. The asterisk indicates a statistically significant difference from Col-0 determined by Student’st-test (P<0.05). Shown is the representative of two independent experiments. (c) Cell morphology of abaxial epidermal cells in the fifth true leaves of Col-0,mos1–6andmad1–2at 4 weeks. Scale bar, 50 μm. (d) Distribution of different cell sizes in Col-0,mos1–6andmad1–2. Figure 6: MOS1 and MAD1 affect endopolyploidization in an opposite manner. ( a , b ) Ploidy levels in the first pair of leaves from ( a ) the wild-type Col-0, mos1–6 and mos1–4 and ( b ) Col-0, mad1–1 and mad1–2 . The error bars indicate s.d. determined from three replicates. The asterisk indicates a statistically significant difference from Col-0 determined by Student’s t -test ( P <0.05). Shown is the representative of two independent experiments. ( c ) Cell morphology of abaxial epidermal cells in the fifth true leaves of Col-0, mos1–6 and mad1–2 at 4 weeks. Scale bar, 50 μm. ( d ) Distribution of different cell sizes in Col-0, mos1–6 and mad1–2 . Full size image We subsequently determined whether or not Arabidopsis SAC components have a role in regulating endopolyploidization ( Fig. 6b ). The two mad1 mutants exhibited reduced endopolyploidization compared with the wild type. At 3-week-old stage, the ploidy profile from 2C to 32C were 7, 24, 53, 15 and 1% in mad1–1 and 8, 28, 51, 12 and 1% in mad1–2 , compared with 5, 19, 51, 23 and 1% in Col-0. Correspondingly, the ploidy indices were 3.02 for Col-0, 2.88 for mad1–1 , and 2.79 for mad1–2 . Therefore, the mad1 mutants had significantly reduced endopolyploidization compared to Col-0. The decrease of the 16C proportion and the reduction of ploidy index were not observed in the mad1 plants at one week old but was evident at 2, 3 and 4 weeks old when the wild type had a drastic increase of the 16C proportion in the leaves ( Supplementary Fig. 5a–c ). Therefore, the Arabidopsis SAC component MAD1 has a regulatory role in endopolyploidization. Since endopolyploidization is generally correlated with the cell size [26] , [27] , we analysed the cell size of abaxial epidermal cell of the fifth true leaf in mos1–6 and mad1–1 at 4 weeks. Visual inspection suggested that mos1–6 had more, while mad1–2 had fewer expanded pavement cells compared with the wild type ( Fig. 6c ). We further categorized the cells into five groups according to their sizes. The mos1–6 mutant had more cells in the two largest size groups, while the mad1–2 mutant had more cells in the second smallest size group compared with Col-0 ( Fig. 6d ). Therefore, the mos1 and mad1 mutations both affect cell sizes, probably due to their effects on endopolyploidization. MAD1 and MAD2 affect MOS1 -regulated endopolyploidization To investigate the interaction of MOS1 with MAD1 in endopolyploidization control, we generated double mutants between mad1–1 and mos1–6 . The double mutant mos1–6 mad1–1 had a ploidy profile of 44% 8C, 27% 16C and 2% 32C, similar to the wild type (45% 8C, 26% 16C and 1% 32C) but different from mos1–6 (34% 8C, 43% 16C and 5% 32C) or mad1–1 (49% 8C, 18% 16C and 1% 32C; Fig. 7a ). Correspondingly, the ploidy index was 2.91 in mos1–6 mad1–1 , similar to 2.91 in the wild-type Col-0 and in between 2.80 in mad1–1 and 3.17 in mos1–6 ( Fig. 7a ). These data indicate that MOS1 and MAD1 antagonistically regulate endopolyploidization. 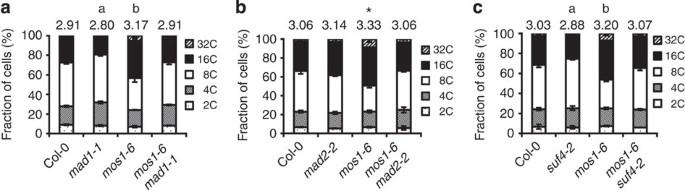Figure 7: Interaction ofMOS1withMAD1,MAD2andSUF4in endopolyploidization modulation. Ploidy levels in the first pair of leaves analysed by flow cytometry from (a) wild-type Col-0,mad1–1,mos1–6andmos1–6 mad1–1; (b) Col-0,mad2–2,mos1–6andmos1–6 mad2–2; and (c) Col-0,suf4–2,mos1–6andmos1–6 suf4–2. Each number above the column indicates the ploidy index of the genotype. The error bars indicate s.d. determined from three replicates. The asterisk indicates a statistically significant difference from Col-0 determined by Student’st-test (P<0.05). The letters a and b indicate statistically significant differences to different extents from Col-0 determined by Student’st-test (P<0.05). Figure 7: Interaction of MOS1 with MAD1 , MAD2 and SUF4 in endopolyploidization modulation. Ploidy levels in the first pair of leaves analysed by flow cytometry from ( a ) wild-type Col-0, mad1–1 , mos1–6 and mos1–6 mad1–1 ; ( b ) Col-0, mad2–2 , mos1–6 and mos1–6 mad2–2 ; and ( c ) Col-0, suf4–2 , mos1–6 and mos1–6 suf4–2 . Each number above the column indicates the ploidy index of the genotype. The error bars indicate s.d. determined from three replicates. The asterisk indicates a statistically significant difference from Col-0 determined by Student’s t -test ( P <0.05). The letters a and b indicate statistically significant differences to different extents from Col-0 determined by Student’s t -test ( P <0.05). Full size image We also analysed the potential role of MAD2 in endopolyploidization control, and did not find significant change of cell ploidy level in the first pair of leaves of the mad2–2 plants at 3 weeks ( Fig. 7b ). However, the mad2 mutation appeared to suppress the endopolyploidization defect in mos1–6 ( Fig. 7b ). The double mutant mos1–6 mad2–2 had a ploidy profile of 2C to 32C at 6, 19, 42, 30 and 3%, which was in contrast with the mos1–6 profile of 7, 16, 28, 40 and 9% but similar to the wild-type profile of 7, 16, 43, 31 and 2%. Overall, the ploidy indices were 3.06 in Col-0, 3.14 in mad2–2 , 3.33 in mos1–6 and 3.06 in mos1–6 mad2–2 . Therefore, MOS1 might inhibit MAD2 to influence endopolyploidization. SUF4 affects MOS1 -regulated endopolyploidization As SUF4 mediates flowering time control in mos1 , we determined whether or not it also mediates the regulation of endopolyploidization in mos1 as well. Ploidy distribution in the first pair of leaves was analysed for Col-0, suf4–2 , mos1–6 and mos1 suf4 at 3 weeks. The suf4–2 single mutant had a slightly reduced ploidy level than Col-0, with 49% 8C and 23% 16C compared with 44% 8C and 29% 16C in Col-0. The mos1 suf4 mutant had a reduced ploidy level than mos1–6 , with 42% 8C, 32% 16C and 3% 32C compared with 29% 8C, 39% 16C and 7% 32C in mos1–6 ( Fig. 7c ). Correspondingly, the ploidy indices were 3.03 in Col-0, 2.88 in suf4–2 , 3.20 in mos1–6 and 3.07 in mos1–6 suf4–2 . Therefore, the suf4–2 mutation largely suppressed the endopolyploidization defect in mos1–6 and the functions of MOS1 in both endopolyploidization and flowering time are dependent on SUF4 . In contrast, the flc-3 mutation, which suppressed the late flowering in mos1 , did not suppress the enhanced endopolyploidization in mos1 . The flc-3 mutant had a ploidy distribution similar to the wild-type Col-0, and the mos1–6 flc-3 double mutant had a profile similar to that of mos1–6 ( Supplementary Fig. 6 ). Therefore, the late flowering phenotype is unlikely the cause of enhanced endopolyploidization in the mos1 mutant. MAD1 and SUF4 co-regulate flowering and endopolyploidization To investigate whether or not MAD1 -regulated flowering time and endopolyploidization are dependent on SUF4 , we introduced the suf4–2 mutation into the mad1–2 mutant. The double mutant suf4–2 mad1–2 had a similar early flowering phenotype to mad1–2 ( Fig. 8a ), and no FLC expression was detected in the double mutant as in the suf4–2 mutant ( Fig. 8b ). At bolting, the double mutant mad1–2 suf4–2 had nine rosette leaves similar to mad1–2 , compared with 13 rosette leaves in Col-0 and suf4–2 ( Fig. 8c ). The mad1 and suf4 single mutants each had a reduction in endopolyploidization, and their double mutant suf4–2 mad1–2 had a similar reduction in endopolyploidization. Ploidy indices were 2.92 in Col-0, 2.74 in suf4–2 , 2.70 in mad1–2 and 2.62 in suf4–2 mad1–2 double mutant ( Fig. 8d ). Although the double mutant had a slightly more reduced ploidy index than the single mutants, the two mad1 and suf4 mutations did not have additive or synergistic effects on the ploidy level, suggesting that MAD1 and SUF4 regulate endopolyploidization through a common pathway rather than two parallel pathways. 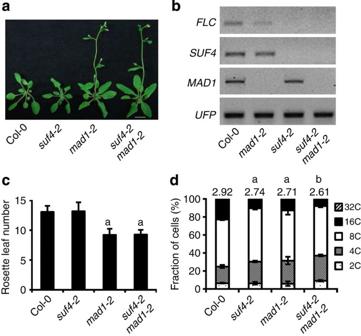Figure 8: MAD1 and SUF4 regulate flowering time and endopolyploidization. (a) Morphology of Col-0,suf4–2,mad1–2andsuf4–2 mad1–2grown for 4 weeks under constant light. Scale bar, 1 cm. (b) RT-PCR analysis ofFLC,SUF4andMAD1expression in the above genotypes. (c) Flowering time measured by rosette leaf numbers at bolting in Col-0 (n=24),suf4–2(n=26),mad1–2(n=27) andsuf4–2 mos1–2(n=28) grown under constant light. (d) Ploidy levels in the first pair of leaves from the wild-type Col-0,suf4–2,mad1–2andsuf4–2 mad1–2analysed by flow cytometry. Shown are mean values and s.d. (error bars) of each ploidy level from three replicates. The letters a and b indicate statistically significant differences at different extents from Col-0 determined by Student’st-test (P<0.05). Figure 8: MAD1 and SUF4 regulate flowering time and endopolyploidization. ( a ) Morphology of Col-0, suf4–2 , mad1–2 and suf4–2 mad1–2 grown for 4 weeks under constant light. Scale bar, 1 cm. ( b ) RT-PCR analysis of FLC , SUF4 and MAD1 expression in the above genotypes. ( c ) Flowering time measured by rosette leaf numbers at bolting in Col-0 ( n =24), suf4–2 ( n =26), mad1–2 ( n =27) and suf4–2 mos1–2 ( n =28) grown under constant light. ( d ) Ploidy levels in the first pair of leaves from the wild-type Col-0, suf4–2 , mad1–2 and suf4–2 mad1–2 analysed by flow cytometry. Shown are mean values and s.d. (error bars) of each ploidy level from three replicates. The letters a and b indicate statistically significant differences at different extents from Col-0 determined by Student’s t -test ( P <0.05). Full size image In this study, we identified three regulators of endopolyploidization in Arabidopsis : MAD1 , MOS1 and SUF4 . Although the plant homologues of SAC components have been implicated in spindle checkpoint control through protein localization studies, this is the first time a plant SAC component is genetically demonstrated to have a role in regulating cell cycle and, in particular, endocycle. In yeast and animals, functional SAC provides an anaphase waiting signal and arrests cell cycle at M phase until all kinetochores are correctly attached. Loss of SAC function may lead to aneuploidy in cancer cells as chromosomes mis-segregate before they are properly attached to the kinetochores [28] , [29] . Here we found a reduction of endopolyploidization in the Arabidopsis mad1 mutant compared with the wild type. This reduced endopolyploidization in mad1 could result from an accelerated completion of the M phase and consequently a reduced opportunity for the transition to endopolyploidization ( Supplementary Fig. 7a ). Detailed cytological analyses may reveal defects in endoreduplication or endomitosis [30] in the mad1 mutants. As the completion of M phase is regulated by SAC in yeasts and animals, this effect of the mad1 mutation on endopolyploidization suggests a similar function of SAC components in plants. Therefore, the decision to complete mitosis or go into endopolyploidization can be influenced by the activity of MAD1 which potentially holds cell cycle at the M phase. In yeasts and animals, MAD1 activity is dependent on its interaction with and recruitment of MAD2 that directly controls the onset of mitosis [30] , [31] . Here we found a physical interaction between MOS1 and MAD2 but not between MOS1 and MAD1. We propose that the Arabidopsis MOS1 is a modulator of SAC activity. MOS1 may compete with MAD1 for interacting with MAD2 and hence inhibit the activity of SAC ( Supplementary Fig. 7a ). In the mos1 mutants, MAD2 is more readily recruited by MAD1 to form functional SAC to inhibit mitosis and promote endopolyploidization. This model is supported by the suppression of endopolyploidization defect in the mos1 mutant by the mad2 and mad1 mutations. A detailed analysis of the dynamics of MAD1, MAD2 and MOS1 during cell cycle and chromosomal behaviour in their mutants will provide further insight on the regulation of endopolyploidization by homologues of SAC components in plants. SUF4 is involved in the modulation of endopolyploidization by MOS1 and SAC components. SUF4 could interact with MOS1, MAD1 and BUB3.1 (ref. 8 ). The loss of SUF4 function reduces endopolyploidization, revealing a new function of SUF4 other than flowering time control. Furthermore, the role of MOS1 and MAD1 in endopolyploidization is dependent on SUF4 as the suf4 mutation suppressed the increased endopolyploidization of mos1 , while the suf4 mad1 double mutant behaves similarly to the single mutants of suf4 and mad1 . It is possible that MAD1 and SUF4 function together to promote endocycle, while MOS1 inhibits endopolyploidization through its binding with MAD2 and/or SUF4 to compete with MAD1 ( Supplementary Fig. 7a ). Another process both MOS1 and MAD1 regulate is the flowering time. FLC is a central regulator of flowering time integrating intrinsic and environmental signals. The mos1 mutants have an upregulation of FLC expression and consequently a late flowering phenotype, both of which can be suppressed by the suf4 mutation ( Figs 3 and 4 ). MOS1 is a nuclear protein and it is associated with the FLC promoter demonstrated by the ChIP experiment. MOS1 itself does not have apparent DNA-binding motifs, so it may become associated with DNA by its interaction with transcription factor SUF4. We propose that MOS1 directly interacts with and inhibits SUF4 to negatively regulate the expression of FLC and therefore to promote flowering ( Supplementary Fig. 7b ). MAD1 may also regulate flowering time through its direct interaction with SUF4, which is supported by the genetic interactions among mad1 , suf4 and FRI . The mad1 suf4 double mutant has the same early flowering phenotype as mad1 , while the mad1 FRI flowered earlier than FRI where SUF4 is recruited by FRI to activate FLC transcription [14] . The full activity of SUF4 may require a functional MAD1 that either forms a complex with SUF4 or modifies SUF4 activity ( Supplementary Fig. 7b ). Further biochemical and genetic studies on the interaction between MAD1 and SUF4 and the FLC locus is needed to vigorously test this model. It is unexpected that SUF4 is also involved in endopolyploidization regulation at least in mutants of mos1 . Since the endopolyploidization defect of mos1 is not dependent on FLC , SUF4, assuming having a transcriptional role, might have additional binding target besides its known target FLC gene. The CYCD3;1 gene could be a candidate for the SUF4 target as its decreased or elevated expressions were reported to promote or reduce endopolyploidization, respectively [32] , [33] , and its expression was correlated with endopolyploidization level in mos1 , mad1 and suf4 mutant combinations ( Supplementary Fig. 8 ). However, no SUF4-binding motif [14] could be identified in the potential regulatory region (4 kb upstream and 2 kb downstream of the coding region) of the CYCD3;1 gene. In addition, CYCD3;1 is a critical and specific factor for the G1 to S phase transition [34] that does not appear to overlap with the proposed function time of SAC. Therefore, CYCD3;1 is likely a marker gene reflecting the change of endopolyploidization but not a direct regulatory target of SUF4. Further investigation of the binding sites of SUF4 in mos1 coupled with transcriptome analysis might reveal the target of SUF4 in endopolyploidization control. That MOS1, MAD1 and SUF4 regulate both endocycle and flowering time raises the question whether or not regulation of one process is a consequence of another. The introduction of flc mutation in mos1 did not alter the endocycle phenotype of mos1 , indicating that endocycle control is not mediated by FLC or flowering time. It is reported that the triple l-o-f mutant cycd3;1–3 exhibited delayed flowering time [33] , suggesting that cell cycle defects can lead to flowering time change. However, the direct binding of SUF4 to the FLC promoter region argues against an indirect regulation of flowering time through altered endopolyploidization. Rather, a co-regulation of flowering time and endocycle might be conferred by MOS1, MAD1 and SUF4. In addition to its role in endocycle and flowering time control, MOS1 is a negative regulator of plant immunity via enhancing the expression of the R gene SNC1 . Recent studies revealed an effect of altered cell cycle progression on plant defense responses against bacterial pathogens. The overexpression of negative regulators of the APC complex, UVI4 and OSD1 , enhances disease resistance against virulent bacterial pathogen by upregulation of R genes including SNC1 (ref. 35 ). Increased nuclear DNA content was observed in leaf cells during infection by bacterial pathogen, suggesting an involvement of endocycle modulation either in defense or susceptibility responses [36] . It is therefore possible that the downregulation of SNC1 expression in mos1 mutants is due to a perturbed cell cycle progression. However, the suppression of the endocycle defect in mos1 by suf4 did not affect the expression level of SNC1 ( Supplementary Fig. 9 ), suggesting that endopolyploidization defect in mos1 is not the cause of altered SNC1 expression. The effects on disease resistance by other cell cycle defects if any in mos1 are yet to be determined. In sum, the Arabidopsis SAC component MAD1 regulates endopolyploidization and flowering time, and SUF4 is involved in these two functions ( Supplementary Fig. 7 ). MOS1 antagonizes the MAD1 activity through its interaction with SUF4 and/or MAD2, and likely serves as a fine modulator of SAC activities. This study reinforces the notion that there is a larger regulation on different processes in plants including growth, flowering time and defense responses [37] . The interaction among MOS1, MAD1 and SUF4 is likely one of the mechanisms for coordinating different processes in response to intrinsic and environmental cues. Plant materials and pathogen tests Seeds of mos1–4 (Salk_126709), mad1–1 (SALK_039008), mad1–2 (Salk_073889) and suf4–2 (SALK_093449) [24] were obtained from the Arabidopsis Biological Research Center (ABRC). For morphological phenotyping and Agrobacterium -mediated transformation, plants were grown at 22 °C under constant light with 50% humidity. For pathogen growth tests, plants were grown under a 12-h light condition and were dip-inoculated at 2 weeks [19] , [38] , [39] . Map-based cloning The sbo3 bon1 double mutant in Col-0 was crossed with bon1–2 SNC1 , which has a functional Col-0 allele of SNC1 introgressed into bon1–2 in Ws. Bulked segregation analyses performed on a DNA pool of 30 mutant plants by about 30 SSLP and CAPS markers [40] identified a linkage of sbo3 to the marker ciw11 on chromosome 4. Further single-nucleotide polymorphism markers were generated by using the website http://msqt.weigelworld.org/ , and 1,450 wild type-like plants were used for fine mapping. Plasmid construction All of the genomic DNA fragments or complementary DNA (cDNA) sequences were first cloned into pDONR221 vector by BP reactions following the manufacture’s instruction (Life Technologies, cat. #11789-020). These entry vectors were recombined with different destination vectors by LR reactions (Life Technologies, cat. #11791-020). Primers used for plasmid construction are listed in Supplementary Table 1 . A genomic fragment of MOS1 from 2.6 kb upstream of the ATG start codon to 30 bp after the ATG was cloned into to the gateway destination vector pGUS1-GW [41] to generate the reporter gene construct. The 10 kb of genomic fragment used to complement the mos1–6 mutation contains the 2.6-kb sequences upstream of the start codon, the coding region, and the 1.5-kb downstream of the TAA stop codon. This fragment was cloned into pGUS1-GW. For the p35S::GFP:MOS1 construct, the MOS1 genomic DNA was cloned into pGWB406 destination vector containing a GFP [42] . Y2H and BiFC For Y2H analysis, cDNAs of gene of interest were cloned into pDEST-GADT7 and pDEST-GBKT7 (ref. 43 ) and assays were performed following the user manual of Matchmaker Gold Yeast Two-Hybrid System (Clontech Laboratories, Inc.). For BiFC analysis, SUF4 cDNA was cloned into the destination vector pSPYNE-35S GW [44] and MOS1 cDNA and MAD1 cDNA were cloned into the destination vector pSPYCE-35S GW [44] . These constructs were transformed into Nicotiana benthamiana via the Agrobacterium strain GV3101 together with gene silencing inhibitor P19 (ref. 21 ). The expression of proteins in the BiFC assay was detected by western blot with proteins extracted and boiled in 1 × SDS–polyacrylamide gel electrophoresis sample buffer. RNA expression analysis Total RNA from 3-week-old seedlings was extracted by Trizol Reagent (Life Technologies, cat. #15596-026) following the manufacturer’s instruction. RNA (30 μg) per sample was separated by gel electrophoresis, and blotted membranes were hybridized with 32 P-labelled DNA probes [19] . For PR1 and SNC1 , the full-length sequence and the first exon of the coding region were used as probes, respectively. qRT-PCR was conducted by following the manufacture’s protocol of FastStart universal SYBR Green Master (Roche). Primers for FLC , CYCD3;1 and the reference gene ubiquitin family protein [17] , [45] are listed in Supplementary Table 1 . ChIP-qPCR analysis ChIP analysis was performed by using Arabidopsis protoplasts [46] overexpressing the MOS1 gene. The MOS1 cDNA was cloned into the pSATN1-GW vector, which was modified from pSAT6-EGFP-N1 vector [47] . Protoplasts were isolated from Col-0 and suf4–2 seedlings, respectively, and the pSATN1-MOS1 construct was transformed into the protoplasts [48] . Protoplasts were then collected at 20 h after transformation, and chromatins were cross-linked with 1% formaldehyde at room temperature for 10 min followed by neutralization with glycine. IP experiments were carried out with anti-GFP monoclonal antibodies (Life Technologies, cat. #A-11120) at a concentration of 6.7 × 10 −3 mg ml −1 (ref. 49 ). PCR primers for different regions of the FLC gene [23] are listed in Supplementary Table 1 . Ploidy measurement Each sample for ploidy measurement was collected from two plants grown under constant light for 3 weeks. The first and second true leaves from these two plants were chopped in ‘Aru’ buffer and filtered by CellTrics 30 μm filter (Partec North America, Inc. Cat. # 04-0042-2316 ) [50] . The nuclei solutions were stained with propidium iodide and measured in a BD Accuri C6 flow cytometer [51] . Ploidy distribution was calculated from more than 5,000 nuclei. Three replicates were analysed for each sample. Every experiment was repeated independently at least twice. The representative data are shown in figures. Ploidy index (PI) was calculated by the formula: PI=(%2C nuclei × 1)+(%4C nuclei × 2)+(%8C nuclei × 3)+(%16C nuclei x4)+(% 32C nuclei × 5). How to cite this article: Bao, Z. et al . Endopolyploidization and flowering time are antagonistically regulated by checkpoint component MAD1 and immunity modulator MOS1. Nat. Commun. 5:5628 doi: 10.1038/ncomms6628 (2014).